A molecular explanation for the recessive nature ofparkin-linked Parkinson’s disease Mutations in the park2 gene, encoding the RING-inBetweenRING-RING E3 ubiquitin ligase parkin, cause 50% of autosomal recessive juvenile Parkinsonism cases. More than 70 known pathogenic mutations occur throughout parkin, many of which cluster in the inhibitory amino-terminal ubiquitin-like domain, and the carboxy-terminal RING2 domain that is indispensable for ubiquitin transfer. A structural rationale showing how autosomal recessive juvenile Parkinsonism mutations alter parkin function is still lacking. Here we show that the structure of parkin RING2 is distinct from canonical RING E3 ligases and lacks key elements required for E2-conjugating enzyme recruitment. Several pathogenic mutations in RING2 alter the environment of a single surface-exposed catalytic cysteine to inhibit ubiquitination. Native parkin adopts a globular inhibited conformation in solution facilitated by the association of the ubiquitin-like domain with the RING-inBetweenRING-RING C-terminus. Autosomal recessive juvenile Parkinsonism mutations disrupt this conformation. Finally, parkin autoubiquitinates only in cis , providing a molecular explanation for the recessive nature of autosomal recessive juvenile Parkinsonism. Parkinson’s disease (PD) is a neurodegenerative disorder that arises from the loss of dopaminergic neurons in the substantia nigra of the midbrain. Typical symptoms include bradykinesia and loss of motor control. In addition to sporadic PD, mutations in six different genes lead to heritable forms of the disease. In particular, homozygous and compound heterozygous mutations in the gene encoding parkin ( PARK2 ) cause 50% of autosomal recessive juvenile Parkinsonism (ARJP) cases resulting in early-onset PD [1] . Parkin is a RING-inBetweenRING-RING (RBR) E3 ubiquitin ligase involved in the ubiquitination of substrate proteins [2] , [3] and mitochondrial mitophagy [4] , [5] . The hallmark of RBR ligases is the presence of two RING (Really Interesting New Gene) domains (RING1 and RING2), separated by an inBetweenRING (IBR) domain ( Fig. 1a ). The family includes the human homologue of the Drosophila Ariadne (HHARI/ARI1), androgen-receptor-associated protein 54, haem-oxidized IRP2 ubiquitin ligase 1 (HOIL-1), HOIL-1-interacting protein (HOIP) and Dorfin [2] , [3] . Parkin also contains an inhibitory N-terminal ubiquitin-like domain (Ubl) (ref. 6 ). Pathogenic mutations leading to ARJP include numerous deletions, truncations and point mutations that occur throughout parkin, but cluster in the Ubl and RING2 domains [7] , [8] . 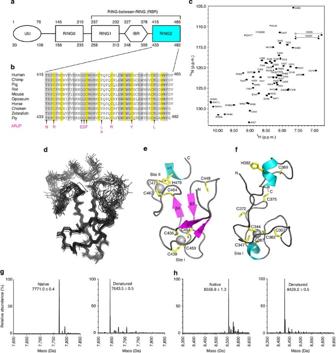Figure 1: Sequence alignment, structure and metal analysis of parkin RING2 domain. (a) Domain structure of parkin showing the C-terminal RING1, IBR and RING2 domains found in all RBR E3 ligase proteins. The ubiquitin-like (Ubl) and RING0 domains are specific to the parkin E3 ligase. Residue numbering is shown for both the human (top) andD. melanogaster(bottom) parkin sequences. (b) Multiple sequence alignment of the RING2 domain for parkin orthologues. Sequence numbers are indicated for the human andD. melanogasterspecies only. Conserved (grey) and cysteine/histidine (yellow) residues are highlighted. Substitutions that contribute to ARJP in the parkin RING2 domain are shown below the sequences (magenta). (c) Assigned 600 MHz1H–15N HSQC spectrum of13C,15N-labelled parkin RING2 (500 μM in 20 mM Tris–HCl, 120 mM NaCl, 1 mM DTT, pH 7.25), labelled using the one-letter amino acid code and residue number according to theD. melanogasterparkin sequence. (d) Superposition of the 20 lowest energy solution structures of parkin RING2 (residues 430–482, backbone r.m.s.d. 0.82±0.17 Å). (e) Ribbon structure of parkin RING2 showing β-strands β1 (T433–P435), β2 (P442–E444), β3 (H451–V453) and β4 (E462–C464), and helix α1 (M476–W480). Side chains for Zn2+-coordinating residues are shown in yellow. (f) Structure of the HHARI RING2 (ref.35) (PDB accession code1WD2) showing different zinc occupancy and fold compared with parkin (e). Deconvoluted mass spectra for native and denatured parkin RING2 (g), and native and denatured HHARI RING2 (h). The mass differences of 127.5 Da (g) and 128.4 Da (h) indicate the presence of two bound Zn2+ions in the native proteins. Raw data are found inSupplementary Figure S2. Structures were visualized using Pymol (PyMOL Molecular Graphics System, Version 1.5.0.4 Schrödinger, LLC). Figure 1: Sequence alignment, structure and metal analysis of parkin RING2 domain. ( a ) Domain structure of parkin showing the C-terminal RING1, IBR and RING2 domains found in all RBR E3 ligase proteins. The ubiquitin-like (Ubl) and RING0 domains are specific to the parkin E3 ligase. Residue numbering is shown for both the human (top) and D. melanogaster (bottom) parkin sequences. ( b ) Multiple sequence alignment of the RING2 domain for parkin orthologues. Sequence numbers are indicated for the human and D. melanogaster species only. Conserved (grey) and cysteine/histidine (yellow) residues are highlighted. Substitutions that contribute to ARJP in the parkin RING2 domain are shown below the sequences (magenta). ( c ) Assigned 600 MHz 1 H– 15 N HSQC spectrum of 13 C, 15 N-labelled parkin RING2 (500 μM in 20 mM Tris–HCl, 120 mM NaCl, 1 mM DTT, pH 7.25), labelled using the one-letter amino acid code and residue number according to the D. melanogaster parkin sequence. ( d ) Superposition of the 20 lowest energy solution structures of parkin RING2 (residues 430–482, backbone r.m.s.d. 0.82±0.17 Å). ( e ) Ribbon structure of parkin RING2 showing β-strands β1 (T433–P435), β2 (P442–E444), β3 (H451–V453) and β4 (E462–C464), and helix α1 (M476–W480). Side chains for Zn 2+ -coordinating residues are shown in yellow. ( f ) Structure of the HHARI RING2 (ref. 35 ) (PDB accession code 1WD2 ) showing different zinc occupancy and fold compared with parkin ( e ). Deconvoluted mass spectra for native and denatured parkin RING2 ( g ), and native and denatured HHARI RING2 ( h ). The mass differences of 127.5 Da ( g ) and 128.4 Da ( h ) indicate the presence of two bound Zn 2+ ions in the native proteins. Raw data are found in Supplementary Figure S2 . Structures were visualized using Pymol (PyMOL Molecular Graphics System, Version 1.5.0.4 Schrödinger, LLC). Full size image RING E3 ligases function by recruiting both a ubiquitin-loaded E2 enzyme and a substrate to catalyse the transfer of ubiquitin. Parkin was originally thought to be a subclass of the canonical RING E3 enzymes, as early studies showed that the RING1 and RING2 domains could each recruit E2-conjugating enzymes, including UbcH7 (UBE2L3), UbcH8 (UBE2L6) and UbcH13/Uev1a [9] , [10] , [11] , [12] , [13] , and lead to autoubiquitination [10] , [11] . Numerous studies show that the RBR domains of parkin, HOIP and HHARI are sufficient for ubiquitination [14] , [15] , [16] . However, the ubiquitination activity of parkin is modulated by its Ubl domain ( Fig. 1a ), proposed to render parkin in an autoinhibited state [6] , [17] . ARJP mutations in the Ubl domain result in constitutively active parkin that is capable of autoubiquitination [6] . Such mutants are unstable in cells, often only detectable in the presence of proteasome inhibitors [6] , [18] . In contrast most C-terminal mutations, particularly those found in RING2, abolish ligase activity [11] , [18] , [19] , [20] , [21] , [22] , [23] , [24] , [25] , [26] . Studies with HOIP and HHARI suggest that RBR ligases form a thiolester intermediate between a cysteine in the RING2 domain and ubiquitin [14] , [15] , [27] . By this mechanism, the RING1 module recruits the E2~ubiquitin complex, whereas RING2 acts as a true catalytic domain performing the transthiolation reaction [14] , [15] , [27] by transferring ubiquitin to a substrate, in a manner analogous to the homologous to E6AP C terminus (HECT)-type ligases [28] . Both parkin and HOIP can catalyse ubiquitin conjugation in the absence of an E2 enzyme [14] , [19] . The loss of the RING1 domain of parkin, thought to be essential for E2 recruitment, does not result in a loss of ligase activity [19] , [25] . Parkin RING2 mutants are catalytically dead in the absence or presence of E2s, whereas mutations outside of RING2 retain both E2-dependent and -independent catalytic activity [24] . These insights suggest that the RING2 of RBR ligases is a catalytic entity that can function in the absence of an E2 enzyme. The mechanism of RBR ligase-catalysed ubiquitin transfer is poorly understood, partly because of a lack of biophysical and structural data on these enzymes. Structures of Ubl domains from parkin and HOIL-1, and the IBR of parkin and HOIP (PDB 2CT7), are available [29] , [30] , [31] , [32] , [33] , [34] . However, little structural data exist for any RBR RING2 domain that would support a catalytic role, identify potential catalytic residues needed to catalyse transthiolation, or identify how this domain might differ from conventional RING E3 ligases. The only available structure of the HHARI RING2 domain shows a loosely organized structure containing a single zinc ion [35] compared with typical RING proteins that possess two metal ions. Although potentially interesting, the HHARI RING2 structure cannot be reconciled with available functional data. Further, the structure sheds little insight on the function of the parkin RING2 domain and how ARJP-causing mutations contribute to the loss of E3 ligase activity. The opposing effects of different mutations in the Ubl and RING2 domains on parkin activity presents an enigma for understanding the loss-of-function phenotype associated with recessive PD. To understand how inhibitory and catalytic domains function in both wild-type parkin and in the disease context, we carried out an extensive biophysical and biochemical characterization of parkin and mutants in solution. We determined structures of the parkin RING2 and IBR–RING2 domains, revealing that the RING2 is neither a canonical RING E3 ligase nor an E2-recruiting module. We find that RING2 is catalytic, identify catalytic residues and show that pathogenic mutations in RING2 perturb the catalytic environment. We show that the tertiary structure of native parkin is dependent on the interaction of the Ubl domain with the RBR region and is disrupted by pathogenic mutations within the N-terminal domain. Finally, we find that constitutively active mutant parkin autoubiquitinates in cis , and not in trans , thereby providing a molecular rationale for the homozygous nature of ARJP. Parkin RING2 is distinct from canonical RING E3 ligases In addition to the characteristic RING1, RING2 and IBR domains, parkin contains N-terminal Ubl and RING0 (ref. 36 ) domains ( Fig. 1a ). We used the RING2 region from Drosophila melanogaster (A417–G482; Fig. 1b ), because it resulted in improved solubility compared with the human protein (residues A398–V465). Numerous studies show that loss of D. melanogaster parkin recapitulates characteristics of PD [37] , [38] . In addition, ARJP variants are conserved between species with the exception of T455 (P437 in human). Initial characterization of fly parkin RING2 by 1 H– 15 N heteronuclear single quantum coherence (HSQC) spectroscopy ( Fig. 1c ) and analytical ultracentrifugation ( Supplementary Fig. S1 ) shows the domain is monomeric and well-folded, but with a disordered N terminus (A417–I429). The solution structure of parkin RING2 shows a well-defined globular fold (root mean squared deviation (r.m.s.d.) 0.82 Å) comprising two pairs of antiparallel β-strands (β1, T433–P435; β2, P442–E444; β3, H451–V453; and β4, E462–C464) and a one-turn C-terminal α-helix (M476–W480) ( Fig. 1d and Supplementary Table S1 ). Two Zn 2+ -binding sites are present comprising residues in the β1–β2 and β3–β4 loops (Site I: C436, C439, C454 and C459) and the loop after β4 and α1 (Site II: C464, C467, C475 and H479). A single cysteine residue (C449; C431 in human) is exposed on the β2–β3 loop, which, according to chemical-shift analysis, was not oxidized or involved in Zn 2+ coordination ( Supplementary Table S2 ). This residue is conserved in all parkin orthologues ( Fig. 1b ) and other RBR sequences. The parkin RING2 structure clearly reveals two Zn 2+ ions coordinated in a linear arrangement consistent with observations that full-length parkin can accommodate eight Zn 2+ ions (that is, two Zn 2+ ions per RING0, RING1, IBR and RING2 domains) [36] . Disagreement exists for the Zn 2+ -coordinating ability of RBR proteins, as the structure of HHARI RING2 shows a single bound Zn 2+ and several non-coordinating cysteine residues [35] ( Fig. 1f ). Substitutions of cysteine residues in parkin render the protein inactive [23] , [24] . Given the importance for the Zn 2+ ion coordination in canonical E3 ligases and cysteine residues in parkin on its function, we used native-state mass spectrometry to identify the metal–ion stoichiometry of the RING2 domains for both parkin and HHARI. Our analyses reproducibly showed that the mass differences between native and denatured states of parkin and HHARI RING2 ( Fig. 1g and Supplementary Fig. S2 ) corresponded to those expected for two Zn 2+ ions, indicating both RING2 domains bind two Zn 2+ ions in their native states. We next used nuclear magnetic resonance (NMR) spectroscopy to reconcile the zinc-binding differences between our data and the previously solved structure of HHARI RING2 (ref. 35 ). The well-dispersed nature of the 1 H– 15 N HSQC spectrum of HHARI RING2 ( Supplementary Fig. S3 ) indicates the protein is well-folded. Analysis of Cα and Cβ chemical shifts for HHARI RING2 reveal that seven cysteines are involved in Zn 2+ coordination ( Supplementary Table S2 ), including C372, C375 and C389 that appear unstructured in HHARI ( Fig. 1f ) but form a well-defined metal centre (Site II) in parkin ( Fig. 1e ). The NMR and mass spectral data clearly show that parkin, HHARI and, probably, all related RBR RING2 domains require the coordination of two Zn 2+ ions for correct folding. The RING2 domain lacks features required for E2 recruitment Comparison of parkin RING2 with canonical RING E3s ( Fig. 2 ) reveals little similarity in protein fold. Parkin RING2 displays a sequential Zn 2+ ion coordination ( Fig. 2a ) where the first and second cysteine pairs and the third and fourth cysteine/histidine pairs act as metal–ion ligands. In contrast, canonical RING E3 ligases, such as TRAF6 or BRCA1, adopt a cross-brace coordination motif [39] , [40] ( Fig. 2c ), using the first and third pairs of cysteines and the second and fourth pair of cysteine/histidine residues. This difference in coordination leads to a more elongated structure for the parkin RING2 domain compared with the more compact fold of canonical RING domains. These structural differences indicate that the RING2 function will not parallel that of canonical RING E3 ligases. 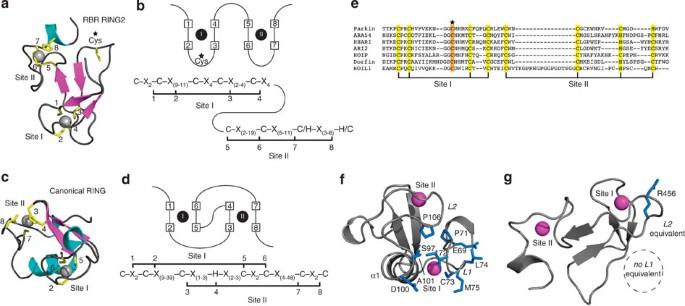Figure 2: RING2 domain of parkin and other RBR E3 ligases do not recruit E2 enzymes. Parkin RING2 defines a novel structure common to RBR ubiquitin ligases that are unable to recruit E2 enzymes. The structures and schematic representations of (a,b) RBR RING2 (parkin) and (c,d) RING (TRAF6, PDB 3HCS) domains showing differences in Zn2+coordination and consensus sequences. (e) Alignment of the RING2 domains of RBR ligases showing residues predicted to coordinate Zn2+(yellow) based on the parkin RING2 structure and the proposed catalytic cysteine conserved in all sequences (orange). (f) Key residues and elements used for E2 recruitment by the canonical RING E3 ligase TRAF6 are found in two loops (L1,L2) formed through Zn2+coordination that are absent in (g) parkin RING2. The structures are oriented using the loops involved in Zn2+coordination for TRAF6 site II and parkin RING2 site I, which exhibit the closest structural similarity. Figure 2: RING2 domain of parkin and other RBR E3 ligases do not recruit E2 enzymes. Parkin RING2 defines a novel structure common to RBR ubiquitin ligases that are unable to recruit E2 enzymes. The structures and schematic representations of ( a , b ) RBR RING2 (parkin) and ( c , d ) RING (TRAF6, PDB 3HCS) domains showing differences in Zn 2+ coordination and consensus sequences. ( e ) Alignment of the RING2 domains of RBR ligases showing residues predicted to coordinate Zn 2+ (yellow) based on the parkin RING2 structure and the proposed catalytic cysteine conserved in all sequences (orange). ( f ) Key residues and elements used for E2 recruitment by the canonical RING E3 ligase TRAF6 are found in two loops ( L1 , L2 ) formed through Zn 2+ coordination that are absent in ( g ) parkin RING2. The structures are oriented using the loops involved in Zn 2+ coordination for TRAF6 site II and parkin RING2 site I, which exhibit the closest structural similarity. Full size image In contrast to the structural dissimilarity with RING E3 ligases, parkin RING2 possesses several features in common with the IBR domains from parkin [32] (PDB accession code 2JMO ) and HOIP (PDB accession code 2CT7 ). With identities below 20%, the sequence of the RING2 domain does not suggest an IBR-fold. However, parkin RING2 superposed well with both IBR structures (backbone r.m.s.d. 2.07 Å and 2.28 Å, respectively) and shares similar Zn 2+ -coordination topology [32] . The surface-exposed cysteine residue (C449) observed in the parkin RING2 structure ( Fig. 2a ) is notably absent in the sequences of other IBR domains [32] . Alignment of the parkin RING2 sequence with other RBR E3s ( Fig. 2e ) shows that all proteins contain conserved cysteine and histidine residues required to coordinate two Zn 2+ ions as observed in the parkin RING2 structure ( Fig. 1e ). This indicates that the architecture and Zn 2+ coordination observed for parkin RING2 is common to all RBR family members. Several structures exist for complexes between RING E3 ligases and E2-conjugating enzymes that allow regions of interaction and function to be identified. For example, the E2:E3 complexes of Ubc13/TRAF6 (ref. 41 ), UbcH5b/cIAP2 (ref. 42 ) and UbcH7/c-Cbl (ref. 43 ) show that two loop regions ( L1 and L2 ) of the RING are integral for E2 recruitment ( Fig. 2f ). Substitutions in these regions compromise the interaction and ubiquitination activity, indicating E2 interaction is necessary for ubiquitin transfer [41] , [42] , [44] . As parkin RING2 is essential for ubiquitination, we reasoned that examining the E2-interacting regions observed in canonical RING E3 ligases might reveal how the RING2 domain in an RBR E3 ligase is involved in a ubiquitination reaction. Using TRAF6 as a template, we find that the RING2 domain lacks the surface and residues typically used by a RING domain to recruit an E2 enzyme as a requisite for ubiquitin transfer. The closest similarity between parkin RING2 and TRAF6 RING domains exists with L2 ( Fig. 2f , r.m.s.d. 1.2 Å for RING2 T434–E444, T455–G458, and TRAF6 V81–K91 and C105–D108). In TRAF6, hydrophobic residues (P71, I72, L74, M75 and P106) within the adjacent L1 and L2 loop regions are used to recruit Ubc13 (ref. 41 ). In particular, a conserved proline (P106 in TRAF6), central to E2 binding, is replaced by a polar side chain group (R456) in parkin RING2. Further, this region lying between the third and fourth chelating cysteine residues from Site I is amongst the poorest conserved in the RBR RING2 sequences ( Fig. 2e ). The most significant difference between the RBR RING2 and canonical RING domain structures occurs for the L1 loop. In parkin RING2, the different Zn 2+ -binding topology places its L1 equivalent on the opposite side of the domain distal from the L2 loop ( Fig. 2g ). These observations indicate that parkin RING2 should be incapable of E2 recruitment using the same binding mode as a canonical E3 RING ligase. To test this hypothesis, we examined the interaction between parkin RING2 and the E2s UbcH7 and UbcH8, which can both facilitate autoubiquitination with full-length parkin [6] , [10] , [11] . As predicted from our structure, we were unable to identify any direct interaction between the IBR or RING2 domains and the E2 enzymes using NMR and isothermal titration calorimetry experiments, even at high concentrations ( Supplementary Fig. S4 ). Our observations demonstrate that parkin RING2, and, by corollary, other RBR RING2 domains are not an E2 recruitment module. Pathogenic RING2 mutations disrupt catalysis The parkin RING2 structure positions a single cysteine (C449 in fly; C431 in human), required for transthiolation and proposed to be catalytic, on the surface of the domain ( Fig. 3a ). To confirm whether this residue is absolutely required for catalysis, we assayed for the formation of a reducible ubiquitin thiolester. We find that active parkin forms a reducible band consistent with the formation of a thiolester ( Fig. 3b , lanes 7 and 8). In contrast, a C431S mutant forms a non-reducible band that is base labile, consistent with an ester adduct ( Fig. 3b lanes 9–11). C431A-parkin does not form either band, indicating that C431 is required for activity and forms a thiolester ( Fig. 3b ), as seen for HHARI and HOIP [15] , [27] . Several ARJP mutations in RING2 (T433N, C436R, G447E, G448D, C449F and C459R in fly; T415N, C418R, G429E, G430D, C431F and C441R in human), which lead to loss of parkin’s E3 ligase activity, have been reported [11] , [18] , [19] , [20] , [21] , [22] , [23] , [24] , [25] , [26] . There are two possible explanations for the loss of ligase activity in these mutants—(i) the substitutions lead to the loss of the integrity of the fold of RING2; or (ii) the substitutions alter the chemical environment of the catalytic cysteine, leading to a loss of catalytic competency. To test these hypotheses, ARJP RING2 substitutions were examined to identify how they might alter the structure of parkin. As expected, C436R- and C459R-substituted proteins were insoluble, consistent with their role in Zn 2+ coordination. All other RING2 proteins were soluble and well-folded as determined by SDS–polyacrylamide gel electrophoresis and NMR analysis ( Supplementary Figs S5 and S6 ), including C449F, the site of the proposed catalytic cysteine. NMR experiments show that most of the substitutions alter the chemical shifts of residues near the unligated cysteine C449 ( Fig. 3a and Supplementary Fig. S6 ). Our observations show that several ARJP substitutions in the RING2 domain likely modify the chemical environment of C449 and interfere with ubiquitin transthiolation. To test this hypothesis, we assayed each of the pathogenic mutants for autoubiquitination activity and observed that all of the mutants exhibited reduced or no activity ( Fig. 3c ). 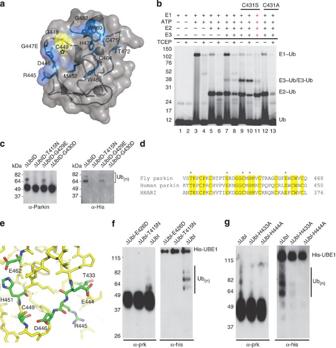Figure 3: Pathogenic mutations in parkin RING2. The structure of parkin predicts catalytic residues conserved between parkin and HHARI. (a) The structure of parkin with the catalytic cysteine highlighted (star) and chemical-shift perturbation experiments show affected residues (blue) in parkin RING2 by the ARJP substitution G447E (magenta). (b) The formation of a reducible parkin~Ub thiolester was monitored using His-SUMO-IBR-R2-parkin. Lanes 1–2 contain E1, Mg2+and Cy5–ubiquitin incubated for 10 min at 37oC. Lanes 3–4 have ATP added for 10 min. Lanes 5–6 have E2 added followed by a further 10-min incubation. Lanes 7–8 have wild-type parkin added. Lanes 9–11 have C431S–parkin added, with NaOH added to lane 11, indicated by red crosses. Lanes 12–13 have C431A–parkin added; ‘−’ and ‘+’ below the line indicate the absence or presence of TCEP. (c) An autoubiquitination assay of folded pathogenic mutants. Parkin–ubiquitin conjugates are detected by western blotting using parkin (left) and His-ubiquitin (right) antibodies. (d) An alignment of the RING2 domains of fly and human parkin, and HHARI. Conserved residues are shaded yellow and the potential catalytic residues are marked with an asterisk. (e) Close-up view of the surface of parkin RING2 with the potential catalytic residues indicated. (f) Autoubiquitination assay of active parkin (ΔUbl) and parkin ΔUbl-E426D. (g) Autoubiquitination assays of active parkin (ΔUbl) and parkin ΔUbl-H433A and ΔUbl-H444A. Infandg, parkin–ubiquitin conjugates are detected by western blotting using parkin (left) and His-ubiquitin (right) antibodies. Figure 3: Pathogenic mutations in parkin RING2. The structure of parkin predicts catalytic residues conserved between parkin and HHARI. ( a ) The structure of parkin with the catalytic cysteine highlighted (star) and chemical-shift perturbation experiments show affected residues (blue) in parkin RING2 by the ARJP substitution G447E (magenta). ( b ) The formation of a reducible parkin~Ub thiolester was monitored using His-SUMO-IBR-R2-parkin. Lanes 1–2 contain E1, Mg 2+ and Cy5–ubiquitin incubated for 10 min at 37 o C. Lanes 3–4 have ATP added for 10 min. Lanes 5–6 have E2 added followed by a further 10-min incubation. Lanes 7–8 have wild-type parkin added. Lanes 9–11 have C431S–parkin added, with NaOH added to lane 11, indicated by red crosses. Lanes 12–13 have C431A–parkin added; ‘−’ and ‘+’ below the line indicate the absence or presence of TCEP. ( c ) An autoubiquitination assay of folded pathogenic mutants. Parkin–ubiquitin conjugates are detected by western blotting using parkin (left) and His-ubiquitin (right) antibodies. ( d ) An alignment of the RING2 domains of fly and human parkin, and HHARI. Conserved residues are shaded yellow and the potential catalytic residues are marked with an asterisk. ( e ) Close-up view of the surface of parkin RING2 with the potential catalytic residues indicated. ( f ) Autoubiquitination assay of active parkin (ΔUbl) and parkin ΔUbl-E426D. ( g ) Autoubiquitination assays of active parkin (ΔUbl) and parkin ΔUbl-H433A and ΔUbl-H444A. In f and g , parkin–ubiquitin conjugates are detected by western blotting using parkin (left) and His-ubiquitin (right) antibodies. Full size image One substitution (T433N) had little effect on the environment of C449; hence, a rationale for the loss of activity is less obvious. In human parkin, the analogous T415N mutation consistently results in an inactive form of parkin regardless of experimental setup [11] , [18] , [19] , [24] , [45] . This threonine is conserved in all parkin orthologues and HHARI ( Figs 1b and 3d ), and rests on the surface of RING2 ~14 Å from the proposed catalytic cysteine. Analysis of the structure revealed a potential catalytic surface hydrogen-bonding network between T433 and a neighbouring glutamate residue (E444; E426 in human) located 3.5 Å from T433, ( Fig. 3e ), which is also conserved in parkin and HHARI. Consistent with this observation, a large chemical shift occurs for E444 in the 1 H– 15 N HSQC spectrum of the T433N-parkin RING2 ( Supplementary Fig. S6a ). This led us to hypothesize that this glutamate could be acting in conjunction with the threonine as a catalytic residue to support the transthiolation reaction by C449. To test this hypothesis, we generated a conservative E426D mutation (human numbering; E444D in fly parkin) in an active form of parkin lacking the N-terminal Ubl domain [6] (ΔUbl, Fig. 3f ). We find that in contrast to ΔUbl–parkin, ΔUbl–E426D is not active for autoubiquitination, further supporting the notion that the RING2 domain is a catalytic entity. In addition to the catalytic cysteine, H451 exhibits a conformation and protonation state consistent with a catalytic role. To test whether H451 (human H433) could act as the proton shuttle between C449 and E462 (human E444), we conducted autoubiquitination assays using H433A and E444A substitutions. Both of these substitutions are unable to support ubiquitination ( Fig. 3f ). Taken together, the structure and subsequent assays reveal the existence of a hydrogen-bonding network involving T433, E444, H451, E462 and semi-conserved R445 and D446 ( Fig. 3e ) that supports the catalytic cysteine required for ubiquitination. IBR and RING2 facilitate interaction with RING0 and RING1 To determine the structural relationship between the IBR domain and the catalytic RING2 domain, we analysed both human and fly IBR–RING2 fragments by NMR spectroscopy and mass spectrometry, and determined the solution structure of fly IBR–RING2. Both human and fly IBR–RING2 structures bind a total of four Zn 2+ ions consistent with structures of the isolated IBR and RING2 domains. The IBR–RING2 structure shows that IBR and RING2 domains are each well-folded but separated by a 26-residue flexible linker between the domains ( Fig. 4a and Supplementary Table S3 ). The lack of interaction between the two domains is supported by the absence of interdomain nuclear overhauser effects (NOEs), near identical peak positions when individual domain 1 H– 15 N HSQC spectra are superimposed with that of IBR–RING2 ( Fig. 4d ), and no observable chemical-shift changes in NMR titrations between RING2 and 15 N-labelled IBR domains ( Supplementary Fig. S7 ). The structure also reveals that the IBR and RING2 domains in IBR–RING2 have similar folds to their independent structures ( Fig. 4b ). Analysis of chemical-shift data indicates that fly and human IBR–RING2 utilize analogous cysteine and histidine residues to coordinate two Zn 2+ ions in each domain ( Supplementary Table S4 ). Together, these results indicate that in the context of native parkin the IBR and RING2 domains are not juxtaposed in the structure. 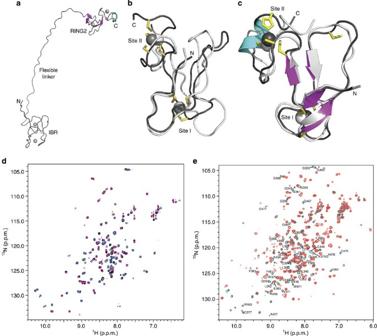Figure 4: The structure of fly IBR–RING2 shows the domains are remote in parkin but interact with RING0 and RING1. (a) Representative ribbon structure of parkin IBR–RING2 showing the flexible linker between the IBR and RING2 domains. (b) The superposition of parkin IBR domains from human (white, PBD accession code 2JMO) and fly (black). (c) The superposition of RING2 domains from fly parkin RING2417–482(white) and fly parkin IBR–RING2342–482(coloured). The two domains adopt similar folds, although the IBR domains do not contain formal β-strands. (d) Superposition of1H–15N HSQC spectra for the fly IBR–RING2 (black contours) with spectra for the individual fly parkin IBR342–402(pink) and RING2417–482(blue) domains. (e) Superposition of1H–15N HSQC spectra for parkin RING0–RING1–IBR–RING2 (red contours) and IBR–RING2342–482(teal contours). The large number of chemical-shift changes indicates that RING0 and RING1 interact with IBR–RING2. Residues in both IBR and RING2 that undergo the largest changes in chemical shift are indicated near their positions from the IBR–RING2 assignment. Figure 4: The structure of fly IBR–RING2 shows the domains are remote in parkin but interact with RING0 and RING1. ( a ) Representative ribbon structure of parkin IBR–RING2 showing the flexible linker between the IBR and RING2 domains. ( b ) The superposition of parkin IBR domains from human (white, PBD accession code 2JMO) and fly (black). ( c ) The superposition of RING2 domains from fly parkin RING2 417–482 (white) and fly parkin IBR–RING2 342–482 (coloured). The two domains adopt similar folds, although the IBR domains do not contain formal β-strands. ( d ) Superposition of 1 H– 15 N HSQC spectra for the fly IBR–RING2 (black contours) with spectra for the individual fly parkin IBR 342–402 (pink) and RING2 417–482 (blue) domains. ( e ) Superposition of 1 H– 15 N HSQC spectra for parkin RING0–RING1–IBR–RING2 (red contours) and IBR–RING2 342–482 (teal contours). The large number of chemical-shift changes indicates that RING0 and RING1 interact with IBR–RING2. Residues in both IBR and RING2 that undergo the largest changes in chemical shift are indicated near their positions from the IBR–RING2 assignment. Full size image To identify how the IBR and RING2 domains might be arranged with respect to the RING0 and RING1 domains in native parkin, we acquired 1 H– 15 N HSQC spectra of fly RING0–RING1–IBR–RING2 ( Fig. 4e ) and compared the data with spectra of IBR–RING2. Unlike the near-perfect superposition of spectra exhibited for the IBR and RING2 domains with the IBR–RING2 fragment, many chemical-shift changes were observed in each of the IBR (that is, D367, V380, V381 and N384) and RING2 (that is, G447, A457, W465 and C475) domains in RING0–RING1–IBR–RING2. This indicates that the environments of these residues in IBR and RING2 are changed by the presence of the RING0 and RING1 domains. The most logical explanation is that the RING0 and/or RING1 domains are interacting with the IBR–RING2 structure forming a more compact arrangement in the protein. Parkin tertiary structure is maintained by the Ubl domain To understand the parkin structure in the context of the native protein, we obtained a molecular envelope of human parkin in solution using small-angle X-ray scattering (SAXS) ( Fig. 5a ). The analysis of the SAXS data, generated from a monodispersed pure sample, indicates that full-length parkin adopts a globular conformation with a radius of gyration of 29.0 Å ( D max 95 Å). Removal of the Ubl domain leads to an extended conformation of parkin ( Fig. 5b ), with a larger radius of gyration (32.0 Å; D max 110 Å) than the 8-kDa larger full-length protein. These observations were validated using sedimentation velocity analysis ( Fig. 5c ) that showed sedimentation coefficients of 4.1 S (parkin) and 3.5 S (ΔUblD–parkin), reflecting the higher mass for parkin. However, the frictional ratio ( f / f 0 ) for ΔUblD–parkin (1.53) was larger than that observed for parkin (1.38). This indicates that ΔUblD–parkin has a more extended conformation, and that in the presence of the Ubl domain parkin adopts a more compact conformation. Activating point mutations in the Ubl domain, R42P, I44A and K48A [6] were also subjected to SAXS analysis and have radii of gyration that were all larger than native parkin (31.8, 30.3 and 29.8 Å, D max 130, 105 and 104 Å, respectively). Despite high-quality data from non-aggregated samples ( Fig. 5d–f ), ab initio modelling cannot be used to interpret the data due to inherent conformational flexibility. Taken together, these data suggest the Ubl associates with the RBR domains in the full-length protein. 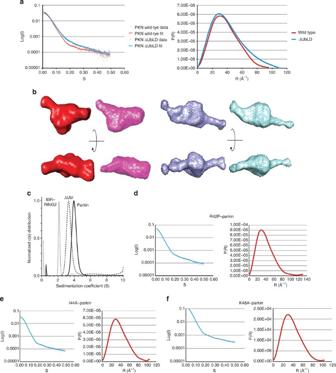Figure 5: The tertiary structure of parkin is maintained by the Ubl. (a) Superposition of the scattering data (left) and distance distribution (right) plots from purified human parkin samples, wild-type (red) and ΔUblD–parkin (blue). The plots show the quality of the data and the radius of gyration. (b) Representative and averagedab initiomodels of wild-type parkin (red/pink) and ΔUbl–parkin (blue/cyan). Two views for each protein are shown rotated 90oabout thexaxis. (c) Sedimentation velocity experiments of parkin, ΔUblD–parkin, and IBR–RING2. All data were analysed using the Lamm equation and fit to a c(s) distribution. Sedimentation coefficients, corrected to 20 °C and in H2O, were determined to be 4.1 S for full-length parkin, 3.5 S for ΔUblD–parkin and 2.2 S for IBR–RING2. Fitted frictional ratios (f/f0) were calculated to be 1.38 for full-length parkin, 1.53 for ΔUbl–parkin and 1.31 for IBR–RING2. Sedimentation velocity experiments were performed at 20 °C using 10–16 μM protein in 25 mM Tris-HCl, 50 mM NaCl, 0.5 mM TCEP, pH 8.0. (d) Scattering data (left) and distance distribution (right) plots for R42P–parkin, (e) I44A–parkin, and (f) K48A–parkin. Figure 5: The tertiary structure of parkin is maintained by the Ubl. ( a ) Superposition of the scattering data (left) and distance distribution (right) plots from purified human parkin samples, wild-type (red) and ΔUblD–parkin (blue). The plots show the quality of the data and the radius of gyration. ( b ) Representative and averaged ab initio models of wild-type parkin (red/pink) and ΔUbl–parkin (blue/cyan). Two views for each protein are shown rotated 90 o about the x axis. ( c ) Sedimentation velocity experiments of parkin, ΔUblD–parkin, and IBR–RING2. All data were analysed using the Lamm equation and fit to a c(s) distribution. Sedimentation coefficients, corrected to 20 °C and in H 2 O, were determined to be 4.1 S for full-length parkin, 3.5 S for ΔUblD–parkin and 2.2 S for IBR–RING2. Fitted frictional ratios ( f / f 0 ) were calculated to be 1.38 for full-length parkin, 1.53 for ΔUbl–parkin and 1.31 for IBR–RING2. Sedimentation velocity experiments were performed at 20 °C using 10–16 μM protein in 25 mM Tris-HCl, 50 mM NaCl, 0.5 mM TCEP, pH 8.0. ( d ) Scattering data (left) and distance distribution (right) plots for R42P–parkin, ( e ) I44A–parkin, and ( f ) K48A–parkin. Full size image Parkin is not a substrate of parkin in trans Our structural data indicate that parkin and parkin mutants form monomers in solution, even at the very high concentrations required for SAXS analysis (up to 0.5 mM). As parkin is reported to be a substrate of parkin, these insights led us to ask whether parkin self-ubiquitination occurs in cis or in trans . To address this question, we first probed the targets of mutant human parkin autoubiquitination by mass spectrometry and identified a conserved site at K349, located within the IBR domain ( Supplementary Fig. S8 ). The IBR–RING2 is sufficient for autoubiquitination activity of parkin [19] , [25] , suggesting that IBR–RING2 is a plausible candidate substrate of full-length mutant parkin. Furthermore, at 17-kDa, IBR–RING2 is easily distinguishable from full-length parkin (52 kDa), or parkin lacking the Ubl domain (46 kDa). The pathogenic mutation T415N in RING2 results in well-folded but inactive protein ( Fig. 3f and Supplementary Fig. S6 ) and, therefore, we used IBR–RING2–T415N as a model substrate for parkin to distinguish between cis and trans autoubiquitination. In contrast to the mutants themselves, IBR–RING2–T415N is not ubiquitinated by any of the active parkin mutants ( Fig. 6a ), even in the presence of a large excess of ‘substrate’ ( Fig. 6b ). To rule out that IBR–RING2–T415N simply does not contain a recognition site for parkin, we expressed and purified full-length haemagglutinin (HA)-tagged T415N–parkin ( Fig. 6c ). Again, even at high concentrations full-length parkin is not a substrate of active parkin. Taken together, these data show that parkin autoubiquitinates in cis , and not in trans. 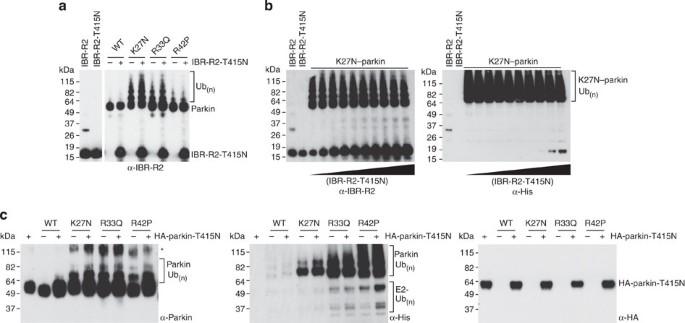Figure 6: Parkin is not a substrate of parkin intrans. (a) Ubiquitination assay using IBR–RING2–T415N (IBR–R2–T415N) as a substrate. Each parkin species point mutation is assayed in the absence (−) or presence (+) of substrate. The first lane shows wild-type active IBR–RING2, the second lane shows the inactive mutant. Parkin–ubiquitin conjugates are detected by western blotting using a parkin antibody. (b) K27N–parkin is assayed for activity towards IBR-R2-T415N with increasing substrate concentration. Parkin–ubiquitin conjugates are detected by western blotting using parkin (left) and His-ubiquitin (right) antibodies. (c) Ubiquitination assay using full-length HA–parkin–T415N as a substrate. Parkin–ubiquitin conjugates are detected by western blotting using parkin and His-ubiquitin antibodies. Unmodified HA-parkin-T415N is detected using HA antibodies. The asterisk denotes a non-specific band. Figure 6: Parkin is not a substrate of parkin in trans . ( a ) Ubiquitination assay using IBR–RING2–T415N (IBR–R2–T415N) as a substrate. Each parkin species point mutation is assayed in the absence (−) or presence (+) of substrate. The first lane shows wild-type active IBR–RING2, the second lane shows the inactive mutant. Parkin–ubiquitin conjugates are detected by western blotting using a parkin antibody. ( b ) K27N–parkin is assayed for activity towards IBR-R2-T415N with increasing substrate concentration. Parkin–ubiquitin conjugates are detected by western blotting using parkin (left) and His-ubiquitin (right) antibodies. ( c ) Ubiquitination assay using full-length HA–parkin–T415N as a substrate. Parkin–ubiquitin conjugates are detected by western blotting using parkin and His-ubiquitin antibodies. Unmodified HA-parkin-T415N is detected using HA antibodies. The asterisk denotes a non-specific band. Full size image There are several classes of E3 ligases, including the RING, U-box and HECT E3s. HECT E3 ligases form a catalytic intermediate via a thiolester with the C terminus of ubiquitin before transferring it to a substrate protein [28] , [46] . In contrast, the RING and U-box E3 ligases function primarily as scaffolds by orienting the E2~ubiquitin thiolester complex and target protein for ubiquitin transfer [47] . Recently, the RBR ligases were proposed to function as a hybrid between the HECT and RING ligases that can also form a catalytic thiolester intermediate [14] , [15] , [27] . In this study we set out to understand the RBR ligase parkin and its domains both in detail, and in the broader context of the whole protein. We determined the structure of parkin RING2 to decipher how this domain might account for the unique RING/HECT hybrid mechanism. We show that parkin RING2 adopts a different fold and Zn 2+ -coordination topology than its RING namesake that likely exists for all RBR ligases. RING2 lacks key residues required for E2/RING interactions, which, in combination with our isothermal titration calorimetry experiments showing no interaction with either UbcH7 or UbcH8, reinforces that RING2 is not an E2 recruitment domain. Likewise, recent observations that parkin IBR–RING2 is capable of E2-independent ubiquitination [19] supports the notion of this RING2 domain having different structural features and activity than canonical RINGs. A key observation from the RING2 structure is the location of a solvent-exposed cysteine that is absolutely conserved in all RBR-containing E3 ligases. This cysteine is perfectly poised to accept an ubiquitin molecule, be it from an E1 or an E2 enzyme, and perform a transthiolation reaction. Clearly, RING2 is the true catalytic domain for the RBR ligases that is not dependent on interacting with an E2 enzyme. Consistent with this, there are numerous ARJP mutations that affect the RING2 domain, not only point mutations but also truncations and deletions that lead to the loss of the RING2 fold [16] ( http://www.molgen.ua.ac.be/PDmutDB ). Understanding the regulation of E3 ubiquitin ligases has become increasingly important in the ubiquitin field. A prime example is the autoinhibited state of the Cullin-RING ligases that can be alleviated by the conjugation of the ubiquitin-like protein NEDD8 to the extreme C terminus of the Cullin, thus increasing the mobility of the Rbx1/ROC1 RING E3 protein for guiding an E2~ubiquitin complex to successfully transfer its ubiquitin cargo to a substrate [48] . Interestingly, several RBR ligases have been recently shown to use autoinhibition to regulate their ubiquitination activity [6] , [14] , [15] , a regulatory mechanism also employed by HECT E3s [49] . There are many aspects of parkin function that are poorly understood, including the structural basis of parkin regulation by a variety of post-translational modifications, and how different E2s impact on parkin activity [10] , [11] , [17] . However, our findings that an affected copy of parkin does not ubiquitinate an unaffected copy suggest a unifying ‘loss-of-function’ rationale for parkin mutations, whereby mutations in the catalytic domain lead to a catalytically inactive parkin, whereas ‘activating’ mutations in the inhibitory domain lead to ubiquitination and subsequent degradation. Our structural analyses in solution combined with biochemical data suggest that in a heterozygous scenario, only the mutant copy of parkin is affected. If the mutation is inactivating, only the mutant copy loses function, and if the mutation is activating only the mutant copy is destroyed. Wild-type parkin is not preyed upon by mutant parkin and remains functional. Our data also provide a molecular rationale for the existence of non-homozygous ARJP sufferers who have compound heterozygous mutations. Protein expression and purification All domains from D. melanogaster PARK2 were cloned into a modified pGEX-6P-2 vector having an N-terminal GST tag and TEV cleavage site (ENLYFQ). Site-directed mutagenesis was used to create all substitutions in parkin RING2. The full length (residues 1–465), ΔUbl (residues 77–465), IBR–RING2 (residues 321–465) domains and substituted proteins from human PARK2 were cloned, expressed and purified as described previously [6] . The RING2 domain of HHARI (residues 325–396) was synthesized by DNA 2.0 (Menlo Park, CA, USA) and cloned into the pGEX-TEV vector. GST-tagged constructs were transformed into Escherichia coli BL21(DE3)-RIL (Stratagene) and grown in Luria broth supplemented with 500 μM ZnCl 2 at 37 °C until OD 600 reached 0.8. Expression was induced with 1 mM isopropylthiogalactoside at 16 °C for 20 h. For 13 C/ 15 N-labelled proteins, cells were grown similarly in M9 media supplemented with 15 NH 4 Cl (1 g l −1 ), 13 C 6 -glucose (2 g l −1 ) and 500 μM ZnCl 2 . Purification used GSTrap FF columns (GE Healthcare) before and following TEV cleavage. Protein solubility experiments Isopropylthiogalactoside-induced overnight cultures (10 ml) were collected and resuspended in 20 mM Tris-HCl, 120 mM NaCl, 5 mM dithiothreitol (DTT), pH 7.4 (1 ml), sonicated for 20 s and centrifuged at 16,000 g for 5 min. The cleared supernatant was separated and the pellet was resuspended in 2% SDS. The preinduction, postinduction, supernatant and pellet samples were then heated in SDS-loading buffer with 5 mM DTT, run on a 16.5% SDS–PAGE gel and stained with Coomassie Brilliant Blue R-250 dye. Metal-binding experiments using mass spectrometry Zinc ion content was assessed by mass spectrometry as previously described [36] . Samples were dialysed twice against 120 mM ammonium acetate pH 7.4, with a final exchange against 10 mM ammonium acetate to remove sodium adducts. Mass spectrometry was performed in positive-ion mode on a Q-TOF Micro mass spectrometer (Waters) with Z -spray source. Denatured proteins were prepared by mixing the native samples with acetonitrile and formic acid (5%) in a 50:50 ratio. Data showed the following masses; fly parkin RING2 C449S (MW calc 7643.6 Da, MW obs (native) 7771.99 Da, MW obs (denatured) 7643.47 Da), human HHARI RING2 C357S (MW calc 8428.2 Da, MW obs (native) 8556.56 Da, MW obs (denatured) 8428.15 Da), human parkin IBR–RING2 (MW calc 16095.34 Da, MW obs (native) 16346.39 Da, MW obs (denatured) 16093.80 Da), fly parkin IBR–RING2 (MW calc 15589.6 Da, MW obs (native) 15842.06 Da, MW obs (denatured) 15588.65 Da), human parkin ΔUbl (MW calc 42834.53 Da, MW obs (native) 43342.07 Da, MW obs (denatured) 42836.07 Da) and fly parkin ΔUbl (MW calc 42470.8 Da, MW obs (native) 42974.25 Da, MW obs (denatured) 42472.0 Da). Isothermal titration calorimetry experiments The interaction of human or D. melanogaster parkin IBR, RING2 or IBR–RING2 with either UbcH7 or UbcH8 was probed by isothermal titration calorimetry using an iTC 200 Microcalorimeter (GE Healthcare). Sample cells contained 30–50 μM of the appropriate parkin domain, and 10 × sample cell concentration in the injection syringe of either UbcH7 or UbcH8. All samples were buffered using 50 mM HEPES, 200 mM NaCl and 250 μM TCEP (tris-(2-carboxyethyl)phosphine) at pH 8.0. Injections of 1.5 μl were dispensed with a 5-s addition time and a spacing of 250 s, with a total of 20 injections at 18 °C. The stirrer speed was 1,000 r.p.m. NMR spectroscopy and structure calculations NMR data were collected using 15 N- or 13 C/ 15 N-labelled parkin domains (100–500 μM) and HHARI RING2 (400 μM) at 25 °C using a Varian Inova 600 MHz NMR spectrometer equipped with a triple resonance probe and z-field gradients. Data were processed using NMRPipe [50] and were analysed using NMRViewJ [51] . Structures were calculated using manual and automatic NOE assignments and dihedral angular restraints (ϕ,Ψ) from TALOS+ (ref. 52 ) incorporated into the programme CYANA [53] . The standard CYANA protocol was used with default settings, involving eight cycles of structure generation and refinement (100 structures per round). Cysteine residues involved in Zn 2+ coordination were identified using Cα and Cβ chemical shifts [54] . The protonation state of histidine residues was determined from Cδ chemical shifts [55] . Initial structures were calculated in the absence of any Zn 2+ -ion restraints so as to not bias the fold of the domain. Following this, zinc atoms were added using virtual linkers. Restraints between the atom pairs Zn–Sγ, Sγ–Cβ, (His Nε2)–Sγ and Sγ–Sγ were imposed to maintain tetrahedral geometry around the zinc ion as previously described [32] . The final 50 structures were water refined using a modified force field in Xplor-NIH [56] . The 20 structures with the lowest NOE energies were chosen as representative of the calculation. Mass spectrometric identity of autoubiquitination sites Ubiquitination experiments were carried out in 50 mM HEPES pH 8.0, 2 mM DTT and 5 mM MgCl 2 containing 5 mM ATP, 200 nM UBE1, 4 μM UbcH7, 16 μM His6-ubiquitin and 2 μM of either R42P, K48A or ΔUblD. Reactions were incubated at 37 °C for 60 min before addition of LDS sample buffer and β-ME. Boiled samples were resolved by gel electrophoresis and gel bands corresponding to ubiquitinated parkin were subjected to further analysis by LC–MS/MS. In vitro ubiquitination assays Reactions were carried out in a total volume of 25 μl in 50 mM Tris pH 7.5, 2 mM DTT and 5 mM MgCl 2 . His mouse UBE1 virus (6 × ) was a kind gift from Kazuhiro Iwai and was purified as a His fusion using Ni-NTA resin (QIAGEN) affinity chromatography followed by size-exclusion liquid chromatography. UbcH7 was purified as previously described [6] . Ubiquitination components were added as follows: 4 mM ATP, 15 nM UBE1, 1.1 μM UbcH7 and 5 μM His6-ubiquitin. Untagged parkin (0.77–1 μM) was added with or without the stated parkin substrate. IBR–R2–T415N (1 μM) or HA–parkin-T415N (0.77 μM) were added in the respective assays unless otherwise specified. Incubation at 37 °C for 60 min preceded addition of SDS buffer and denaturation by boiling. Samples were resolved by gel electrophoresis and analysed by western blot. Antibodies used for visualization were as follows: anti-parkin (1/5,000, 1A1; IBL), anti-6 × His (1/2,000; GE Healthcare), anti-HA (1/1,000; Mono-HA.11, Covance) and anti-IBR-R2 raised against recombinant IBR-R2 (Pettingill Technology Ltd). Full blots and gel scans are included in Supplementary Fig. S9 where appropriate. Parkin thiolester in vitro ubiquitination assays Cy5-labelled His6-ubiquitin was generated as described [15] . A cysteine residue was inserted between the 6xHis tag and the first methionine by site-directed mutagenesis. Purification was carried out initially on a HiLoad 16/10 Q-Sepharose High Performance column (GE Healthcare) equilibrated in 25 mM Tris, 1 mM EDTA, at pH 8. His6-ubiquitin eluted in the flowthrough was then concentrated and purified further using size-exclusion chromatography. Protein was stored in 50 mM HEPES pH 7.5. Purified protein (1 mg) was incubated at room temperature with one vial of Cy5 Maleimide Mono-Reactive Dye (GE Healthcare) in a 550 μl total reaction volume for 90 min with gentle agitation. Excess dye was removed on a 5 ml HiTrap Desalting column (GE Healthcare) equilibrated in 50 mM HEPES pH 7.5 and 150 mM NaCl. Labelled protein was further purified by size-exclusion chromatography. Reactions were buffered in 50 mM Tris pH 7.5 and contained 2 mM DTT and 5 mM MgCl 2 . Cy5-His6-ubiquitin (1 μM), 2 μM UBE1 and 1 mM ATP were mixed and incubated at 37 °C for 10 min before addition of 10 μM UbcH7, and a further 10 min incubation at 37 °C. 20 μM His-SUMO-IBR-R2, His-SUMO-IBR-R2-C431S or His-SUMO-IBR-R2-C431A-parkin was then added. The native parkin was incubated for only 15 s, C431S was incubated at 37 °C for 1 h, and a sample incubated with 0.15 M NaOH. Reactions were stopped using NuPAGE LDS Sample Buffer (Invitrogen) and were reduced by the addition of TCEP and boiling where indicated. Gels were visualized using an ImageQuant LAS 4000 imaging system. Analytical ultracentrifugation Sedimentation velocity experiments were performed using a Beckman Coulter XL-A analytical ultracentrifuge equipped with an An-60 Ti rotor. Samples (400 μl) were prepared in 25 mM Tris–HCl, 50 mM NaCl and 0.5 mM TCEP pH 8.0, and centrifuged in a double sector cell (1.2 cm) equipped with sapphire windows at 45,000 r.p.m. at 20 °C. Samples were scanned at equal intervals (60 scans total) and the absorbance at 280 nm measured with three replicates averaged per scan. Data were analysed using the programme Sedfit using non-linear regression to determine the frictional ratio ( f / f 0 ) for each species as well as the sedimentation coefficient corrected to 20 °C. All data were fit to an r.m.s.d. equal or less than 0.008. SAXS data collection and processing SAXS data were collected at Synchrotron Soleil; beamline SWING. Samples ranging in concentration from 5 to 25 mg ml −1 were directly passed into the beam from HPLC gel filtration using an Agilent BioSec-3 300 column. Data were collected from the peak(s) comprising the protein of interest, avoiding any aggregates with data for the buffer blank collected before the elution of protein from the column. Initial data processing was undertaken automatically using the FOXTROT software at the beamline. Further processing, using the ATSAS suite (version 2.5.0— http://www.embl-hamburg.de/biosaxs/software.html ), was undertaken using PRIMUS [57] (for initial R g and Kratky plot analysis), GNOM [58] (generation of distance distribution plots) and DAMMIF [59] (generation of ab initio models). Models were converted to Situs format using PDB2VOL (part of the SITUS suite, http://situs.biomachina.org/ ). Figures were produced using CHIMERA [60] followed by superimposition of envelopes. Accession codes : Atomic coordinates and structural restraints have been deposited in the RCSB Protein Data Bank under PDB accession codes 2LWR and 2M48. NMR assignments have been deposited to the Biological Magnetic Resonance Data bank under accession codes 18642 and 18990 . How to cite this article : Spratt, D. E. et al . A molecular explanation for the recessive nature of parkin -linked Parkinson’s disease. Nat. Commun. 4:1983 doi: 10.1038/ncomms2983 (2013).